Electrochemical mechanism of ion current rectification of polyelectrolyte gel diodes Polyelectrolyte gel diodes that are double layers of two oppositely charged polyelectrolyte gels, sandwiched by two symmetric electrodes, are emergent ionic devices. These diodes are designed to rectify ion currents with a physical mechanism that is analogous to conventional semiconductor diodes—the asymmetry in the permeability of ions across the interfaces between the two oppositely charged gels. Here we show that polyelectrolyte gel diodes indeed rectify steady currents with a physical mechanism that is very different from conventional diodes by using a simple electrochemical model; electric currents are limited by electrochemical reactions that are driven by potential drops at electrodes and these potential drops markedly change with changing the direction of applied voltages due to the redistribution of non-reactive counterions, leading to rectified ion currents. This concept is relatively generic and thus may provide insight in the physics of analogous ionic and biomimetic systems that show electrochemical reactions. Diodes show very large electric currents in one direction (forward), but show only very small currents in the opposite direction (reverse), and are used to rectify electric currents in many home electronic appliances. Electric currents in conventional semiconductor p–n diodes are mostly limited by the transports of electrons and holes across the junctions between p-type and n-type semiconductors, where these electric carriers are depleted [1] , [2] . p–n diodes rectify electric currents because the densities of electrons and holes in p-type and n-type semiconductors are already asymmetric [1] , [2] ; electric currents are carried by the majority carriers of each type of semiconductors for forward voltages and by their minority carriers for reverse voltages. Can one design diodes that rectify other types of electric currents, for example, ion currents in electrolyte solutions? Nanochannels of asymmetric shapes were shown to rectify ion currents that are generated by Ag/AgCl electrodes [3] , [4] , [5] , [6] . Polyelectrolyte gel diodes (PGDs) that are the double layers of two oppositely charged polyelectrolyte gels (that are swollen in aqueous solutions), sandwiched by two symmetric metal electrodes, are another type of ionic diodes that rectify ion currents [7] , [8] , [9] , [10] , [11] , [12] , [13] , [14] , [15] , [16] . These diodes are designed to operate with a physical mechanism that is analogous to conventional semiconductor diodes—the asymmetry in the permeability of ions across the interfaces between the two oppositely charged gels [8] , [9] , [10] , [11] , [12] . However, in contrast to p–n diodes, where electrons and holes are the carriers of the entire systems, for the cases of PGDs, electric currents are carried by electrons in the external circuits and are carried by ions in the polyelectrolyte gels; PGDs do not show steady electric currents unless electrons are transferred between electrodes and reactants by electrochemical reactions. Because electrochemical reactions are driven by voltages applied between electrodes and reactants (that are at the surfaces of these electrodes), potential drops at the surfaces of electrodes are key parameters that determine electric currents in PGDs. This situation is very different from the cases of semiconductor p–n diodes, where voltages applied at interfaces between semiconductors and electrodes do not play an essential role in their operations. Recent experiments have shown that salt impurity must be eliminated for PGDs to rectify (steady) ion currents [8] , [9] . This implies that electrostatic potentials, which are generated by the electric charges of polyelectrolyte gels and their counterions (that are not the reactants or products of the electrochemical reactions), play an important role in the operation of PGDs. We thus theoretically analyse electrostatic potentials in PGDs to predict the physical mechanisms involved in the ion current rectification of PGDs by using a simple electrochemical model. Our theory predicts that PGDs rectify ion currents with a physical mechanism that is very different from conventional p–n diodes: for reverse voltages, counterions are recruited from the interface between the two oppositely charged gels to neutralize electric charges that are induced at the electrodes and the electric charges of carrier ions that are produced by electrochemical reactions at the electrodes. The fixed electric charges of the polyelectrolyte gels that are left at this interface generate large potential drops there. These potential drops greatly suppress electrochemical reactions at the electrodes. In contrast, for forward voltages, electric charges on the electrodes and the electric charges of carrier ions are neutralized by the fixed electric charges of polyelectrolyte gels; these fixed charges generate large potential drops at the surfaces of the electrodes and thus enhance electrochemical reactions at these electrodes. Our theory predicts that the conservation of the number of counterions plays a key role in the operation mechanisms of PGDs. Experimentally measuring electrostatic potentials in PGDs would thus advance our understanding of the operational mechanisms of these devices. Our theory is relatively generic and thus may be extended to analogous ionic and biomimetic systems that show electrochemical reactions. Electrochemical model Our models are designed to eliminate the asymmetry of electric currents arising from the specific chemistry of individual experimental systems to highlight the role played by the electric charges of polyelectrolyte gels and their counterions (see Methods for details); without polyelectrolyte gels and their counterions, electric currents are completely symmetric with respect to forward and reverse applied voltages. Because the system is symmetric with respect to the center, z =0, see Fig. 1 , we treat only a half of the system, z >0. The ionic groups of polyelectrolyte gels are essentially immobile (and thus are treated as uniform fixed charges), and, in contrast, their counterions freely diffuse in the entire volume of the system; our model thus extends the treatments of these ions that have been developed in soft matter physics [17] , [18] , [19] , [20] , [21] , [22] , [23] to electrochemical systems. Analogous models are used to treat electrolyzers [13] , [14] , [15] , [24] , [25] and fuel cells [26] , [27] , [28] that use polymer electrolyte membranes. We treat the cases in which counterions are not the reactants or products of electrochemical reactions. Hydrogen and hydroxide ions are produced at the positive and negative electrodes, respectively, due to the electrolysis of water molecules (that are abundant in the system). In these cases, the dynamics of the system is limited by electrochemical reactions at the electrodes. The production rates of hydrogen and hydroxide ions are determined by potential drops at the electrodes and are equal to the fluxes of these ions in steady states; potential drops at the surfaces of the electrodes are key parameters that determine electric currents in PGDs. In the next few sections, we treat the cases in which there is no additional salt (no-salt regime), where the number of each of the positive and negative counterions is conserved. 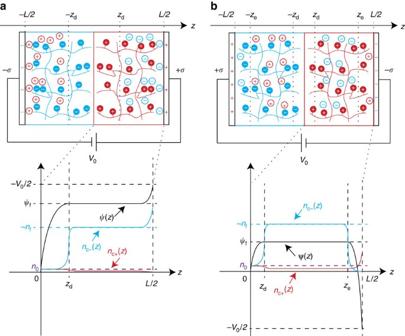Figure 1: Electrostatic potentials in the equilibrium. Polyelectrolyte gel diodes (PGD) are the double layers of two oppositely charged polyelectrolyte gels that are sandwiched by two symmetric electrodes. Experiments have shown that PGDs show very small electric currents for reverse applied voltages (a),V0<0, and show very large electric currents for forward applied voltages (b),V0>0, for the cases in which salt impurity is eliminated8,9. The bottom figures schematically show electrostatic potentialsψ(z) (the black solid curve) and the local densities of positive and negative counterions,nc+(z) andnc−(z), (the red and blue solid curves) in a half of the PGD,z>0, for the cases in which electrochemical reactions at the electrodes are suppressed. The ionic groups of polyelectrolyte gels are treated as uniform fixed electric charges (these charges are shown by + and − with filled circules) and the distributions of their counterions are functions of electrostatic potentials (these counterions are shown by + and − with open circles). PGDs show depletion layers, where counterions are depleted, at the interface region between the two oppositely charged gels, 0<z<zd, and the surfaces of the electrodes,ze<z<L/2. Electrostatic potentialsψ(z) are approximately constantψfin the bulk region of polyelectrolyte gels. Bulk electrostatic potentialsψfare (halves of) potential drops across the depletion layer at the interface between the two gels and thus are generated by the fixed charges of the polyelectrolyte gel in this layer. Figure 1: Electrostatic potentials in the equilibrium. Polyelectrolyte gel diodes (PGD) are the double layers of two oppositely charged polyelectrolyte gels that are sandwiched by two symmetric electrodes. Experiments have shown that PGDs show very small electric currents for reverse applied voltages ( a ), V 0 <0, and show very large electric currents for forward applied voltages ( b ), V 0 >0, for the cases in which salt impurity is eliminated [8] , [9] . The bottom figures schematically show electrostatic potentials ψ ( z ) (the black solid curve) and the local densities of positive and negative counterions, n c+ ( z ) and n c− ( z ), (the red and blue solid curves) in a half of the PGD, z >0, for the cases in which electrochemical reactions at the electrodes are suppressed. The ionic groups of polyelectrolyte gels are treated as uniform fixed electric charges (these charges are shown by + and − with filled circules) and the distributions of their counterions are functions of electrostatic potentials (these counterions are shown by + and − with open circles). PGDs show depletion layers, where counterions are depleted, at the interface region between the two oppositely charged gels, 0< z <z d , and the surfaces of the electrodes, z e < z < L /2. Electrostatic potentials ψ ( z ) are approximately constant ψ f in the bulk region of polyelectrolyte gels. Bulk electrostatic potentials ψ f are (halves of) potential drops across the depletion layer at the interface between the two gels and thus are generated by the fixed charges of the polyelectrolyte gel in this layer. Full size image Electrostatics We first treat relatively simple cases in which electrochemical reactions at the electrodes are suppressed. Counterions are distributed to neutralize the fixed electric charges of polyelectrolytes in the bulk of the gels and are depleted in the regions at the interface between the two gels, 0< z < z d (depletion layers), see Fig. 1 . Electrostatic potentials ψ ( z ) are thus approximately constant in the bulk of the polyelectrolyte gels and show potential drops at the depletion layer and the surface of the electrode owing to excess charges in these regions, see the bottom figure in Fig. 1 and also Supplementary Note 1 (refs 19 , 20 ). Because potential drops ψ f at the interface between the two gels are generated by the fixed charges of polyelectrolyte gels in the depletion layer, these potential drops increase with increasing the thickness z d of the depletion layer. For reverse voltages ( V 0 <0, see Fig. 1a ), potential drops ψ f at the interface between the two gels are relatively sensitive to applied voltages, see Fig. 2 . This is because counterions are recruited from the interface between the two gels to neutralize electric charges on the electrodes and this increases the thickness z d of the depletion layer at this interface. In contrast, for forward voltages ( V 0 >0, see Fig. 1b ), potential drops ψ f at the interface between the two gels are not sensitive to applied voltages, see Fig. 2 . This is because electric charges on the electrodes are neutralized by the fixed electric charges of the polyelectrolyte gels, instead of recruiting counterions from the interface between the two gels; the thickness of the depletion layer is thus not sensitive to applied voltages. 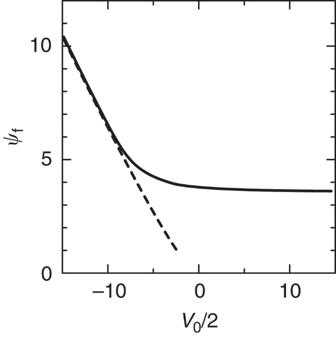Figure 2: Potential drops at the gel–gel interfaces versus applied voltages. Potential dropsψfare shown as functions of the halves of applied voltagesV0/2 (shown in the unit of the thermal voltage) for the cases in which the value of the rescaled thicknessκfLof PGDs is 1.0 × 104, the solid curve. Equations that are used for the calculations are shown inSupplementary Note 7. The broken curve is predicted by using a scaling theory (shown inSupplementary Note 10) for relatively large reverse voltages. Figure 2: Potential drops at the gel–gel interfaces versus applied voltages. Potential drops ψ f are shown as functions of the halves of applied voltages V 0 /2 (shown in the unit of the thermal voltage) for the cases in which the value of the rescaled thickness κ f L of PGDs is 1.0 × 10 4 , the solid curve. Equations that are used for the calculations are shown in Supplementary Note 7 . The broken curve is predicted by using a scaling theory (shown in Supplementary Note 10 ) for relatively large reverse voltages. Full size image Reverse currents in the no-salt regime For reverse applied voltages, V 0 <0, hydrogen ions that are generated at the positive electrodes, z = L /2, diffuse (via the positive polyelectrolyte gel) towards the center z =0 of the system, where these hydrogen ions are associated with hydroxide ions that diffuse from the other side of the system, z <0. The positive charges of hydrogen ions in the bulk of the positive polyelectrolyte gel (where electrostatic potentials are relatively large) are neutralized by negative counterions that are recruited from the interface between the two gels (where electrostatic potentials are relatively small). In a length scale that is larger than the Debye screening length ( ; l B is the Bjerrum length, ~7Å, and n t is the sum of the densities of positive and negative counterions in the bulk of the gels), hydrogen ions are treated as diffusing particles that show short-range repulsive interactions with the second virial coefficient (see Supplementary Note 2 ). In a steady state, the local density of hydrogen ions thus has an approximate form for the bulk of the gel, z d < z < L /2. λ t (≡− D hyd n t / J H ) is a length scale that characterizes the distribution of hydrogen ions (we call it ‘diffusion length’, not to be confused with the usual definition in semiconductor physics [1] ), where D hyd is the diffusion constant of hydrogen (and hydroxide) ions (see also the discussion below equations (9) and (10) in Methods). Equation (1) implies that hydrogen ions are distributed in the entire volume of the gel. In general, the diffusion length is relatively large ( L / λ t <1, for relatively small currents that are treated in our theory). Because the positive charges of hydrogen ions are neutralized by negative counterions, electrostatic potentials are approximately constant ψ f in the bulk of the gel; applied voltages are thus distributed to the interface between the two gels and the surfaces of the electrodes, analogous to the cases of the equilibrium, see the bottom figure, Fig. 1a . However, the values of the thickness z d of the depletion layer and potential drops ψ f across this layer are very different from the cases of the equilibrium (see below). Our theory predicts that very small ion currents are generated in PGDs for reverse voltages V 0 <0, see Fig. 3a . This is because applied voltages that are distributed to the surfaces of the electrodes are very small owing to very large potential drops ψ f that are generated at the interface between the two gels; a very large number of negative counterions are recruited from the interface between the two gels to neutralize the positive charges of hydrogen ions that are distributed in the entire volume of the positive polyelectrolyte gel, see equation (1), and the electric charges of the polyelectrolyte gel that are left at this interface generate large potential drops there. This is in contrast to the cases of the equilibrium, where negative counterions are recruited only to neutralize relatively small electric charges on the electrodes. We here emphasize that potential drops ψ f at the interface between the gels are very sensitive to the magnitudes of reverse currents; the number of hydrogen ions that are accumulated in the bulk of the gel increases with increasing reverse currents, see equation (1), and thus more negative counterions are recruited to neutralize the electric charges of these hydrogen ions. 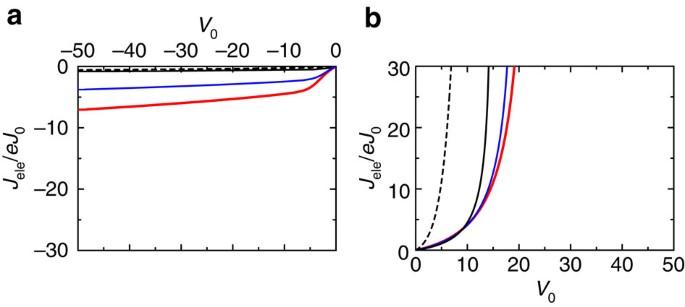Figure 3: Electric currents versus applied voltages without additional salt. Electric current densitiesJele(=eJH=−eJOH) (that are rescaled by exchange current densityeJ0, see Methods) are calculated as functions of applied voltagesV0(in the unit of the thermal voltage) for reverse (a) and forward voltages (b). The number of hydrogen and hydroxide ions that are accumulated in the bulk of the gel increases with decreasing the values ofκfλ0(that is defined by equation (2)). We usedκfλ0=1.0 × 106(black solid curve), 5.0 × 106(blue) and 1.0 × 107(red) for the calculations. The value of (rescaled) gel thicknessκfLis fixed to 1.0 × 104. The equations that are used for the calculations are shown inSupplementary Notes 8 and 9. We used a simple scaling argument (shown in Methods) to predict the (black) broken curve ina. The (black) broken curve inbshows the cases in which all of the applied voltages are distributed to the surfaces of the electrodes. This is also supported by the fact that reverse currents decrease with decreasing the values of a parameter Figure 3: Electric currents versus applied voltages without additional salt. Electric current densities J ele (= eJ H =− eJ OH ) (that are rescaled by exchange current density eJ 0 , see Methods) are calculated as functions of applied voltages V 0 (in the unit of the thermal voltage) for reverse ( a ) and forward voltages ( b ). The number of hydrogen and hydroxide ions that are accumulated in the bulk of the gel increases with decreasing the values of κ f λ 0 (that is defined by equation (2)). We used κ f λ 0 =1.0 × 10 6 (black solid curve), 5.0 × 10 6 (blue) and 1.0 × 10 7 (red) for the calculations. The value of (rescaled) gel thickness κ f L is fixed to 1.0 × 10 4 . The equations that are used for the calculations are shown in Supplementary Notes 8 and 9 . We used a simple scaling argument (shown in Methods) to predict the (black) broken curve in a . The (black) broken curve in b shows the cases in which all of the applied voltages are distributed to the surfaces of the electrodes. Full size image see Fig. 3a , where the number of hydrogen ions that are accumulated in the gel increase with decreasing this parameter, see equation (1) ( n f is the density of ionic groups of polyelectrolyte gels, is an inverse length and J 0 is exchange current density, see also Methods). A scaling theory that is based on the above argument (shown in Methods) predicts that reverse currents scale as , see the black broken curve in Fig. 3a ; reverse currents are thus sensitive to the thickness L of the gels. These results imply that the conservation of the number of counterions plays an essential role in suppressing electric currents in reverse applied voltages. Our results are effective for relatively small applied voltages (for example, the experiments in refs 8 , 9 ), where the dissociations of water molecules by electric fields at the interface between the two gels are negligible [14] , [15] (in practice, the onset of water dissociations is sensitive to the chemical properties of polyelectrolyte gels [16] ). Forward currents in the no-salt regime For forward voltages, V 0 >0, hydroxide ions that are produced by electrochemical reactions at the electrode, z = L /2, diffuse to the center of the system, z =0, via the positive polyelectrolyte gel, see Fig. 1b . The negative charges of hydroxide ions are neutralized by the fixed electric charges of the positive polyelectrolyte gel; a part of negative counterions are released from the positive polyelectrolyte gels. With an argument that is similar to the cases of reverse voltages, one can show that the local density of hydroxide ions has an approximate form in the bulk of the gel (see Supplementary Note 2 ). The diffusion length, λ t (≡− D hyd n t / J OH ), is relatively large also for forward voltages (unless electric currents are very large) and hydroxide ions are distributed in the entire volume of the gel. Because the negative charges of hydroxide ions are neutralized by the electric charges of the positive polyelectrolyte gel, applied voltages are distributed to the interface between the two gels and the surfaces of the electrodes, in a similar manner to the case of the equilibrium, see Fig. 1b . Our theory predicts that electric currents in PGDs increase exponentially with increasing (forward) applied voltages, see Fig. 3b . This is because applied voltages are mostly distributed to the surfaces of the electrode: potential drops at the interface between the two gels are not sensitive to applied voltages because the negative charges of hydroxide ions are neutralized by the fixed charges of the positive polyelectrolyte gel; counterions stay at the interface between the two gels. Moreover, in the bulk region, the positive polyelectrolyte gel releases their negative counterions to neutralize the negative charges of hydroxide ions (we here remind the readers that positive counterions are released from the other side of the system, z <0, with a similar mechanism). Electric charges that are induced at the surface of the electrode are neutralized by these released counterions and the fixed charges of the positive polyelectrolyte gel; these electric charges stabilize the electric double layer that efficiently drop electrostatic potentials at the surface of this electrode. For relatively small applied voltages, V 0 /2< ψ f , electric currents are not very sensitive to the values of λ 0 (where hydroxide ions that are accumulated in the bulk of the gel increase with decreasing λ 0 , see equations (2) and (3)), see V 0 <10 in Fig. 3b . This is because, in these small applied voltages, the number of released counterions is relatively small and thus electric charges at the surface of the electrode are mostly neutralized by the fixed charges of the gel. In contrast, for relatively large applied voltages, electric currents increase with decreasing the values of λ 0 , see V 0 >10 in Fig. 3b . This is because released counterions increase with increasing electric currents and thus reinforce the electrostatic screening of electric charges on the electrodes. We here emphasize that the conservation of the number of counterions plays a key role in the reinforcement of the electrostatic screening by released counterions. Effects of additional salt We have shown that the conservation of the number of counterions plays a key role in the rectification of ion currents in PGDs. We here treat the cases in which a PGD is in a solution of salt ions that are the same chemical species as the counterions of the polyelectrolyte gels of this PGD (salty regime); because this solution serves as the reservoirs of additional salt ions that are indistinguishable from counterions (we here call them salt ions too), the number of counterions (and salt ions) in the PGD is no longer conserved (see Methods). Our theory predicts that electric currents exponentially increase with increasing applied voltages even for reverse voltages, see Fig. 4a (we here refer ‘reverse’ for the direction of applied voltages that is shown in Fig. 1a , V 0 <0, and ‘forward’ for the opposite direction, following the definition in the rest of this paper). This is because, for reverse voltages, the electric charges of hydrogen ions that are generated at the electrode (and the electric charges on this electrode) are neutralized by salt ions that are recruited from the reservoirs, instead of recruiting counterions from the interface between the two gels; potential drops at the interface between the two gels are insensitive to applied voltages. This is an important result that demonstrates that the conservation of the number of counterions plays an important role in suppressing electric currents for reverse applied voltages. 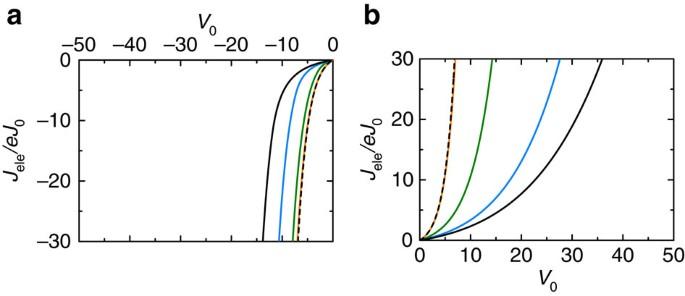Figure 4: Electric currents versus applied voltages with additional salt. Electric current densitiesJele(=eJH=−eJOH) (that are rescaled by exchange current densityeJO) are shown as functions of applied voltagesV0for the cases that forward (a) and reverse (b) voltages are applied to PGDs in solutions of additional salt. We here refer ‘reverse’ for the direction of applied voltages that is shown inFig. 1a, and ‘forward’ for the direction that is shown inFig. 1b, following the definition of the rest of this paper. We calculated for the cases in which the values of rescaled concentrationsns/nfof salt in the reservoir are 0.001 (black solid curve), 0.01 (light brue), 0.1 (green) and 1.0 (orange). The values ofκfλ0and the (rescaled) thicknessκfLof the device are fixed to 1.0 × 106and 1.0 × 104, respectively. The (black) broken curves (both (a,b)) are (rescaled) electric currents for the cases in which all of applied voltages drop at the surfaces of the electrodes (these broken curves almost overlap the orange curves). Figure 4: Electric currents versus applied voltages with additional salt. Electric current densities J ele (= eJ H =− eJ OH ) (that are rescaled by exchange current density eJ O ) are shown as functions of applied voltages V 0 for the cases that forward ( a ) and reverse ( b ) voltages are applied to PGDs in solutions of additional salt. We here refer ‘reverse’ for the direction of applied voltages that is shown in Fig. 1a , and ‘forward’ for the direction that is shown in Fig. 1b , following the definition of the rest of this paper. We calculated for the cases in which the values of rescaled concentrations n s / n f of salt in the reservoir are 0.001 (black solid curve), 0.01 (light brue), 0.1 (green) and 1.0 (orange). The values of κ f λ 0 and the (rescaled) thickness κ f L of the device are fixed to 1.0 × 10 6 and 1.0 × 10 4 , respectively. The (black) broken curves (both ( a , b )) are (rescaled) electric currents for the cases in which all of applied voltages drop at the surfaces of the electrodes (these broken curves almost overlap the orange curves). Full size image For the cases in which the concentration of salt ions in the reservoir is larger than (a half of) the density of electric charges of polyelectrolytes, n s > n f /2, electric currents are symmetric with respect to forward and reverse voltages, see the orange curves in Fig. 4a,b . Indeed, in these cases, all of the applied voltages are distributed to the surfaces of the electrodes, to a good approximation, see the (black) broken curves in Fig. 4a,b . Our theory predicts that electric currents are indeed slightly smaller for forward voltages than reverse voltages for the cases in which the concentrations of salt ions are smaller than (a half) the density of polyelectrolyte charges, n s < n f /2, see Fig. 4a,b . This is because, for reverse voltages, positive charges on the electrode, see Fig. 1a , are neutralized by negative salt ions that are recruited from the reservoir (these salt ions are relatively abundant because of the bulk electrostatic potentials ψ f arising from the positive charges of polyelectrolytes). In contrast, for forward voltages, negative charges on this electrode are mostly neutralized by the fixed charges of the positive polyelectrolyte gel (because the concentrations of salt ions in the reservoir are relatively small); this electrostatic screening is limited by the density n f of the electric charges of the gel. In some cases, electric currents for forward voltages are even smaller than the cases of no-salt regime, see Figs 3b and 4b . This is because, in the salty regime, positive and negative counterions that are released from the polyelectrolyte gels (to neutralize the negative charges of hydroxide ions, see the preceding section) diffuse to the reservoir (that has much larger volumes, but have smaller salt concentrations than the PGD for n s < n f /2) owing to their translational entropy. In contrast, in the no-salt regime, these released counterions remain in the PGD (because the number of counterions is conserved) and thus reinforce the electrostatic screening of electric charges on the electrodes. This demonstrates the fact that the conservation of the number of counterions plays an important role in generating large electric currents in forward voltages. Experimentally, salt impurity is always included in PGDs even when salt ions are not deliberately added. A natural question may be, experimentally, when PGDs operate in the salty regime and when they operate in the no-salt regime. In the salty regime, a PGD is connected with reservoirs that have much larger volume than the PGD; the number of salt ions in the reservoir is practically infinite although the concentration n s of salt ions in this reservoir is finite. For the cases in which the number of additional salt ions in the system is finite (and thus is not connected with the reservoir) and is smaller than the number of electric charges that are to be neutralized by these additional salt ions (the electric charges of hydrogen and hydroxide ions and electric charges on the electrodes), counterions are recruited from the interface between the two gels to neutralize these electric charges; in this case, the conservation of the number of counterions is effective and thus PGDs operate in the no-salt regime. It is thus important to eliminate salt impurity for PGDs to rectify ion currents. This result is indeed in agreement with recent experiments [8] , [9] . Our theory predicts that electric currents in PGDs are rectified by physical mechanisms that are very different from those of conventional semiconductor p–n diodes: for the cases of PGDs, the distribution of electrostatic potentials markedly change with changing the direction of applied voltages because of the redistribution of (non-reactive) counterions. This is in contrast with the cases of p–n diodes, where voltages mostly drop at their p–n junctions for both forward and reverse voltages; these diodes rectify electric currents because the densities of hole and electrons in p-type and n-type semiconductors are already asymmetric. Organic diodes that have the junction of (solid) p-type and n-type semiconducting organic materials [29] , [30] , [31] are operated by injecting carriers (electrons or holes) from the electrodes [31] , [32] , [33] , [34] . At a first glance, one may think these organic diodes are analogous to PGDs because electric carriers in both of the two diodes are brought from the exterior by electron transfer. However, the only electric charges in organic materials are those of carriers and thus voltages are mostly applied to the bulk of organic materials [34] , [35] . This is in contrast to the case of PGDs, where the electric charges of carriers are neutralized by the electric charges of polyelectrolyte gels and their counterions and thus voltages are mostly applied to interfaces; the unique rectification mechanism of PGDs is because of the electrochemical nature of these systems. Critical experimental tests on our theory may advance our understanding of the physical mechanisms involved in the ion current rectification of PGDs. Our theory predicts the following experimentally accessible predictions: first, voltages are mostly distributed to the interfaces between the two gels for reverse voltages and to the surfaces of the electrodes for forward voltages. This prediction may be accessible by using experimental techniques that measure local electric fields, for example, electric field-induced second harmonic generation [32] , and/or techniques that capture the signature of redistribution of counterions, for example, cyclic voltammetry, fluorescence microscopes with charged probes [10] and electrochemical impedance spectroscopy [28] . Second, the asymmetry of electric currents increases (forward currents increase and reverse currents decrease) with decreasing values of , see Fig. 3 and equation (2); κ f λ 0 is thus an important parameter that determines the performance of PGDs (see also Supplementary Discussion ). This prediction is experimentally accessible by systematically changing the density n f of the ionic groups of polyelectrolyte gels and fixing the rescaled thicknesses κ f L of the polyelectrolyte gels to a constant value. We note that the diffusion constant D hyd of hydrogen and hydroxide ions may depend on the density n f of the ionic groups of polyelectrolyte gels for the cases in which this density is very large (see also Methods) [22] . Third, reverse currents scale as the inverse of square of the thickness L of PGDs. This prediction is experimentally accessible by systematically changing the thickness L . Although our theory is relatively generic, this theory is ideally tested by experiments that satisfy the following conditions: first, electrochemical reactions at the electrodes are limited by the rate of these reactions. Our theory may not be effective for the cases in which electrochemical reactions at the electrodes are limited by the transport of reactants (for example, for the cases that counterions are the reactants or products of the electrochemical reactions [10] , [11] , [24] , [25] , [26] , [27] ). Second, polyelectrolyte gels that are used to prepare PGDs are stiff enough; polyelectrolyte gels that do not have enough stiffness may locally collapse to neutralize electric charges on the electrodes [20] , [21] , [36] . The subthreshold behaviours of electric currents for forward voltages in the no-salt regime, see V 0 <10 in Fig. 3b , and the slight asymmetry of electric currents for relatively small salt concentrations in the salty regime, see Fig. 4 , may thus be sensitive to the stiffness of polyelectrolyte gels. Experiments by systematically changing the density of crosslinks of the gels may be useful to understand the latter effects. Third, electric currents are measured in steady states because, otherwise, electric currents may deviate from our predictions due to transient capacitive currents arising from the redistribution of counterions. However, the cases in which these conditions are not satisfied may be treated by using an extension of our theory (and also the variants of PGDs [37] , [38] ). In conclusion, our theory predicts that electrostatic potentials in PGDs markedly change with changing the direction of applied voltages due to the redistribution of non-reactive (counter) ions and this leads to rectified ion currents. These non-trivial behaviours are due to the conservation of the number of these ions. This situation is very different from usual cases of conventional electronics devices, but is relatively generic in electrochemical systems. We thus anticipate that our theory will provide insight in the physics of analogous ionic and biomimetic systems that show electrochemical reactions and is useful to design PGDs and other ionic devices that control ion currents. Polyelectrolyte gels and counterions PGDs are the double layers of two oppositely charged polyelectrolyte gels that are sandwiched by two symmetric electrodes. We treat relatively stiff polyelectrolyte gels that are treated as uniform fixed charges. The ionic groups of the positive and negative polyelectrolyte gels are symmetric ions—these ions have the same properties except for the fact that they have electric charges of the opposite sign, and the densities of the ionic groups of the two gels are both n f . Moreover, positive and negative counterions are also symmetric ions. With these treatments, the system is symmetric with respect to z =0, see Fig. 1 . Both the ionic groups of the polyelectrolyte gels and their counterions are monovalent and thus a simple mean field theory is effective [17] . We treat the cases that the Gouy–Chapman length of these polyelectrolyte gels is smaller than their thickness L /2, where l B (≡e 2 /(4π εT )) is the Bjerrum length, where e is the elementary charge, T is the absolute temperature (in the unit of Boltzmann constant) and ε is the dielectric constant of the polyelectrolyte gels (that are assumed to be uniform in the system). In these cases, electrostatic interactions between the polyelectrolyte gels and their counterions dominate the free energy contributions of the translational entropy of counterions [19] , [20] and thus the electric charges of polyelectrolyte gels are neutralized by their counterions in the bulk region. We treat the cases in which counterions are not the reactants or products of electrochemical reactions at the electrodes. In these cases, the fluxes of positive and negative counterions are zero and thus the local densities of positive and negative counterions are distributed with the Boltzmann distribution that has the form respectively. ψ ( z ) are electrostatic potentials (in the unit of the thermal voltage T / e ) and is determined by the Poisson equation (see below). n 0 are the local densities of positive and negative counterions at z =0 (where electrostatic potentials are zero). e is the base of natural logarithm (not to be confused with italic e that represents the elementary charge). For the cases that there is no additional salt, the number of each of positive and negative counterions is conserved; where we used the fact that the number of negative counterions that enter the region of the negatively charged gel, z <0, is equal to the number of positive counterions in the region of the positively charged gel, z >0, because of the symmetry of the system [18] . n f L/2 is the total number of each of the positive and negative counterions. Electrochemical reactions Hydrogen ions are produced by electrochemical reactions at positively charged electrodes, 2H 2 O→O 2 +4H + +4e − , where the standard electrode potentials (electrostatic potentials that are necessary to induce electrochemical reactions) of these reactions are 1.23 V. Hydroxide ions are produced by electrochemical reactions at negatively charged electrodes, 2H 2 O→H 2 +2OH − −2e − , where the standard electrode potentials of these reactions are 0.83 V. We treat the cases of a PGD that is in equilibrium with the reservoir of water molecules; water molecules are thus not depleted from the system. The rates, at which hydrogen and hydroxide ions are produced by the electrochemical reactions at the electrodes, are treated by using Buttler–Volmer equations that have the form where Δ V are overpotentials (the excess of electrostatic potentials that are applied between the electrode and reactants from standard electrode potentials) and J 0 is exchange current density (the rate of one side, forward or backward, of reactions at the equilibrium, Δ V =0). In practice, exchange current densities J 0 may be sensitive to the electrostatics and chemistry of polyelectrolyte gels and the metals that are used for electrodes [25] , [26] , [27] . Because water molecules in the solvent of polyelectrolyte gels are relatively abundant, compared with products, we neglect backward reactions that produce water molecules; equations (7) and (8) are only effective for Δ V >0 and Δ V <0, respectively. In general, the exchange current densities and standard electrode potentials of the two electrochemical reactions (at the positive and negative electrodes) are somewhat different. We neglect the asymmetry of exchange current densities between these two reactions. Moreover, we neglect standard electrode potentials altogether; hydrogen ions are produced at electrodes, to which positive voltages are applied, and hydroxide ions are produced at electrodes, to which negative voltages are applied. We identify overpotentials Δ V as potential drops at electric double layers at the electrode Δ V = E L/2 / κ f − η 0 , where E L/2 is electric fields at z = L /2 and is an inverse length. The zero of overpotentials η 0 is set to potential drops at the electric double layers for the cases in which applied voltages are zero; this ensures that electrochemical reactions are not driven for zero applied voltages (see also Supplementary Note 3 ; Supplementary Fig. 1 ). With this treatment, ion currents are completely symmetric with respect to forward and reverse applied voltages for the cases in which there are no polyelectrolyte gels and their counterions in the system. This model enables us to demonstrate a generic mechanism of ion current rectification (that does not depend on the specific chemistry of experimental systems) by using a simple model. Transport equations of hydrogen and hydroxide ions Hydrogen and hydroxide ions that are generated at the electrodes, z =± L /2, diffuse to the center of the system, z =0, via the bulk of the polyelectrolyte gels. Hydrogen and hydroxide ions do not show chemical reactions in the bulk of the polyelectrolyte gels and thus the fluxes of these ions are constant in this region (see also ‘association of hydrogen and hydroxide ions’ below). The fluxes of hydrogen and hydroxide ions have the form where the subscripts H and OH indicate hydrogen and hydroxide ions. The first terms of equations (9) and (10) are diffusion currents and the second terms of these equations are drift currents that are driven by electric fields. n H ( z ) and n OH ( z ) are the local densities of hydrogen and hydroxide ions. We used the Einstein relationship to derive equations (9) and (10). We treated hydrogen and hydroxide ions as symmetric ions; this is to highlight the roles played by the electric charges of polyelectrolyte gels and their counterions in the ion current rectification of PGDs. D hyd is the diffusion constant of hydrogen and hydroxide ions (this constant depends on the volume fraction and the density of the ionic groups of polyelectrlyte gels for the cases in which these parameters are relatively large [22] and thus should be measured by separate experiments or predicted by using multiscale modelling [24] , [25] , [26] , [27] , [28] ). For the dilute limit, the values of the diffusion constants of hydrogen and hydroxide ions are 1.27 × 10 −4 and 7.15 × 10 −5 cm 2 s −1 , respectively. The treatments of these equations are shown in Supplementary Notes 2 and 4 . Poisson equation Electrostatic potentials are generated by the electric charges of hydrogen ions, hydroxide ions, the polyelectrolyte gels and their counterions and are derived by using the Poisson equation that has the from where n pol ( z ) is the local density of fixed polyelectrolyte charges; n f for z >0 and − n f for z <0. Association of hydrogen and hydroxide ions Hydrogen and hydroxide ions that are transported to the center of the system, z =0, via the bulk of polyelectrolyte gels are associated at this position with chemical reactions H + +OH − →H 2 O. We assume that the rate constant k ass of these association reactions is relatively large and thus hydrogen and hydroxide ions do not enter the other side of the system; this ensures the continuity of the fluxes of hydrogen and hydroxide ions in the bulk region. The local density of hydrogen and hydroxide ions, n H ( z ) and n OH ( z ), are thus zero at z =0 (the absorbing boundary conditions). Steady states and boundary conditions In steady states, the rates at which hydrogen and hydroxide ions are produced by electrochemical reactions at z =± L /2, the fluxes of these ions, and the rate at which these ions are associated at z =0 are all equal; S H = S OH =− J H = J OH for reverse voltages and S H = S OH =− J OH = J H for forward voltages, see equations (7, 8, 9, 10). Solving these equations and the Poisson equation (11) leads to the local densities of hydrogen and hydroxide ions, n H ( z ) and n OH ( z ), and electrostatic potentials ψ ( z ). We apply the absorbing boundary conditions to the local densities of hydrogen and hydroxide ions at z =0, n H (0)= n OH (0)=0 (see also ‘association of hydrogen and hydroxide ions’ and Supplementary Note 5 for an approximate treatment). We apply two boundary conditions to electrostatic potentials: (i) electrostatic potentials ψ ( z ) are zero at z =0 (because of the symmetry of the system); (ii) electric fields, , are E L /2 (≡− eσ /(ε T )) at z = L /2, where σ is the area density of electric charges that are induced on the electrode at z = L /2 ( σ has the unit of C m −2 ). The boundary condition (i) ensures that electric fields E ( z ) at z =− L /2 are E L/2 (ref. 18 ). We derived electrostatic potentials at z = L /2 (that are indeed the negative of halves of applied voltages, − V 0 /2) as functions of the fluxes of hydrogen and hydroxide ions. We used an approach that was used in refs 19 and 20 to treat these equations (see Supplementary Note 1 ). Main analytical results that are derived by using this approach are shown in Supplementary Notes 6–9 . Additional salt To treat the effects of additional salt, we treat the cases in which PGDs are in contact with the reservoir of salt ions that are the same chemical species as the counterions of polyelectrolytes. Because salt ions in the reservoir and counterions are indistinguishable, the number of counterions is no longer conserved and thus equation (6) is not effective. Moreover, equations (4) and (5) are replaced with respectively [17] , where n s is the concentration of salt ions in the reservoir (and thus is a control parameter). With these expressions, the electrostatic potential in the reservoir is set to zero. The local density of each of the positive and negative salt ions at z =0 is n s because electrostatic potentials there are zero owing to the symmetry of the system [17] , [18] . Bulk electrostatic potentials ψ s have the form , where it is a constant that is determined solely by the concentration of salt ions in the reservoir. Scaling argument for reverse currents For the cases in which the diffusion length λ t is relatively large, the local density of hydrogen ions scales as , equation (1). The total number of hydrogen ions that are distributed in the gel is . Because negative counterions are recruited from the interface between the two gels to neutralize the positive charges of these hydrogen ions, n f z d ≃ N H , the thickness of the depletion layer at this interface is , where the length λ f is defined by D hyd n f /(− J H ). Indeed, for the case of relatively large reverse voltages, λ f ≃ λ t , because the local density of positive counterions is very small in the region of the positive polyelectrolyte gel, n 0 ~0 (this is indeed not the case for forward voltages because of released counterions). Potential drops across the depletion layer (at the interface between the two gels) are . For the cases in which applied voltages are mostly distributed to these potential drops, ψ f ≃ − V 0 /2, the thickness of the depletion layer is . The two expressions of the thickness of the depletion layer lead to . How to cite this article: Yamamoto, T. et al. Electrochemical mechanism of ion current rectification of polyelectrolyte gel diodes. Nat. Commun. 5:4162 doi: 10.1038/ncomms5162 (2014).